Emergent neutrality leads to multimodal species abundance distributions Recent analyses of data sampled in communities ranging from corals and fossil brachiopods to birds and phytoplankton suggest that their species abundance distributions have multiple modes, a pattern predicted by none of the existing theories. Here we show that the multimodal pattern is consistent with predictions from the theory of emergent neutrality. This adds to the observations, suggesting that natural communities may be shaped by the evolutionary emergence of groups of similar species that coexist in niches. Such self-organized similarity unifies niche and neutral theories of biodiversity. Species abundance distributions (SADs) summarize how abundance varies among species and are amongst the most studied descriptors of community structure in ecology. One common approach to plot SADs is to show a histogram of number of species on the y -axis against log-transformed abundance on the x -axis [1] . Over the years, there has been a remarkable proliferation of SAD models [2] , [3] that all, without exception, predict unimodal curves on a log scale. However, there is evidence that SADs may, in fact, be multimodal (for example, Fig. 1 ). For instance, Dornelas and Connolly [4] find a multimodal SAD in coral data collected by extensive sampling around a Pacific island. In this analysis, multimodality is robust to sampling noise, strongly suggesting that the underlying distribution of species abundances genuinely departs from unimodality. Similarly, McGill et al . [3] note that a three-mode distribution best fits the SAD in the Barro Colorado Island tree data set, a survey that has so far only been used to compare models producing classic unimodal curves [5] , [6] . There are several reasons why multiple modes could be regularly 'missed' in SADs. First of all, binning methods are prone to blur such patterns [3] . Also, the common approach that combines data across guilds and/or regions can easily mask multimodality occurring at the local scale [3] , [4] , [7] . More fundamentally, the idea that SADs could be multimodal has been largely overlooked [3] . Dornelas and Connolly [4] recently mentioned possible multimodality in published SADs of communities of trees [3] , [8] , birds [9] , fish [10] , fossil brachiopods [11] , benthos [12] , phytoplankton [13] , [14] , insects [15] and nematodes [15] . We collected some of those data sets and carried out statistical analyses that confirmed multimodality ( Fig. 1b–d ; Supplementary Table S1 for details). Many more data sets remain to be explored, but our overview suggests that multimodal SADs might well be frequent in nature. Obviously, accepting this point of view would mean having to reject every existing SAD theory that assume some level of species symmetry [3] including the classical resource-partitioning models [16] , [17] , models based on stochastic population dynamics [18] and neutral models [19] , [20] , which all yield unimodal curves. As we will demonstrate, emergent neutrality (EN) [21] may be a notable exception, as it predicts multimodal SADs under virtually all conditions. 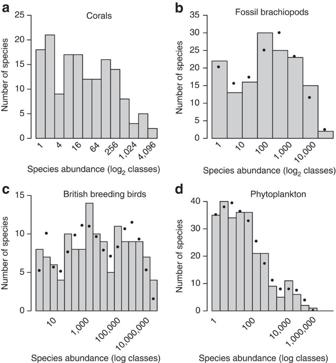Figure 1: Examples of multimodal species-abundance distributions on log scales. (a) Corals around Lizard Island, Great Barrier Reef (modified from Dornelas and Connolly4); (b) Fossil Permian Brachiopods from the Lower Word Formation, Texas (modified from Olszewski and Erwin11); (c) British breeding birds (data compiled by Bakeret al.41); and (d) Carribean phytoplankton (data taken from Margalef42). Abundance is recorded as (a) colonies counted in 275 transects, (b) abundance of species in geological sequence, (c) population size estimates as given by the British Trust for Ornithology (mean values were taken when only size ranges were available), (d) abundance of species estimated from 1,144 of 150 ml-samples taken in the South-East Caribbean Sea. Following the method described extensively by Dornelas and Connolly4we fitted mixtures of one, two and three Poisson lognormal distributions to the data and compared goodness-of-fit, using Akaike information criterion (AIC), Bayesian information criterion (BIC) and the likelihood ratio tests (LRT). The black dots correspond to the best fit. All goodness-of-fit measures suggest the presence of two modes in SAD (b) and two or three modes in the data set (c). AIC and LRT indicate two modes in SAD (d), but the much more conservative BIC did not pick up multimodality in that case. Dornelas and Connolly4analyzed the data set (a) and found three modes in the abundance distribution. Data set (a) is binned in log2abundance classes (1, 2–3, 4–7, 8–15 and so on). SAD (b) is binned in log2abundance classes of width 2, whereas SADs (c) and (d) are binned in log abundance classes of width 1. Note that these different representations are used to show as clearly as possible the underlying modes and have no influence on the result of the statistical analysis itself. Figure 1: Examples of multimodal species-abundance distributions on log scales. ( a ) Corals around Lizard Island, Great Barrier Reef (modified from Dornelas and Connolly [4] ); ( b ) Fossil Permian Brachiopods from the Lower Word Formation, Texas (modified from Olszewski and Erwin [11] ); ( c ) British breeding birds (data compiled by Baker et al . [41] ); and ( d ) Carribean phytoplankton (data taken from Margalef [42] ). Abundance is recorded as ( a ) colonies counted in 275 transects, ( b ) abundance of species in geological sequence, ( c ) population size estimates as given by the British Trust for Ornithology (mean values were taken when only size ranges were available), ( d ) abundance of species estimated from 1,144 of 150 ml-samples taken in the South-East Caribbean Sea. Following the method described extensively by Dornelas and Connolly [4] we fitted mixtures of one, two and three Poisson lognormal distributions to the data and compared goodness-of-fit, using Akaike information criterion (AIC), Bayesian information criterion (BIC) and the likelihood ratio tests (LRT). The black dots correspond to the best fit. All goodness-of-fit measures suggest the presence of two modes in SAD ( b ) and two or three modes in the data set ( c ). AIC and LRT indicate two modes in SAD ( d ), but the much more conservative BIC did not pick up multimodality in that case. Dornelas and Connolly [4] analyzed the data set ( a ) and found three modes in the abundance distribution. Data set ( a ) is binned in log 2 abundance classes (1, 2–3, 4–7, 8–15 and so on). SAD ( b ) is binned in log 2 abundance classes of width 2, whereas SADs ( c ) and ( d ) are binned in log abundance classes of width 1. Note that these different representations are used to show as clearly as possible the underlying modes and have no influence on the result of the statistical analysis itself. Full size image The theory of EN predicts a competition-driven, self-organized evolutionary emergence of groups of similar species [21] . EN implies that species in nature should be organized in clusters where they coexist in essentially the same niche, thereby bridging a gap between niche [22] and neutral theory [20] . A core idea is that there are two different ways for species to coexist, being sufficiently different or being sufficiently similar. The EN model simulates a community of competing species, each characterized by their position on a 'niche axis' [21] . Species that are closer on the niche axis compete more strongly. Species are created randomly along the niche axis and compete with their neighbors, depending on how similar and abundant these are. Each species slowly evolves its position on the niche axis in the direction where it experiences less competition. Although one would expect that the survivors of this evolutionary game would be species that are equally spread out over the niche axis, the surprising result is a pattern of self-organized modes that contain multiple coexisting species [21] ( Supplementary Fig. S1 ). Coexistence of different modes is a straightforward effect of competition avoidance. However, species that are similar enough escape this rule of limiting similarity and may coexist within the modes. In each of the modes, species are almost equivalent—almost neutral—and as no species is clearly superior to another, the process of displacement is very slow. As a consequence, competitive exclusion can easily be prevented by common density-dependent mechanisms that promote stable coexistence. The evolutionary convergence of species towards a same niche seems counter-intuitive. However, it has long been known that as species niches become more closely packed, positions between species can turn into the worst places to be in the 'fitness landscape' and evolutionary convergence between close species may occur [22] . So far, empirical support for EN comes from 'lumpiness' reported in the size distributions of species ranging from phytoplankton and zooplankton to mammals and birds [23] , [24] , [25] . As body size is a major aspect in determining the ecological niche of many organisms [26] , [27] , the existence of such groups of species of similar size suggests clustering in the niche space, as predicted by the theory. Recently, a novel empirical test pointed to EN as the only theory consistent with patterns observed within a real marine phytoplankton community [28] . Further analyses carried out on different communities are now being published [29] , [30] that will ultimately show how common this result is. Here we show that, unlike any other competition or evolution theory, EN predicts the multimodal SADs. To do so, we run the EN model under realistic conditions and compute the corresponding SADs, looking specifically at the presence or absence of multiple modes. In a first simulation, we run the original model without evolution [21] and examine how the abundance of the randomly generated competing species becomes distributed. Although evolution is central in explaining the robustness of EN predictions, this simpler model is sufficient to illustrate how competition affects differently the species' abundances along the niche axis. In natural communities, it is unlikely that the entire niche space is equally suitable [25] , [31] , and resource availability or the intensity of physiological or energetic constraints may vary among externally imposed pre-existing niches. To integrate such heterogeneity, we relax in a second simulation the assumption that all niches are self-organized by organisms, and allow parts of the niche space to be inherently better than others. We implement evolution in this particular simulation to illustrate the key idea of species adapting to pre-existing niches. In a third simulation, we envisage a size-structured community, where the niche of a species is defined by its body size, reflecting many real communities where this is an acceptable approximation [26] , [27] . Larger-bodied species are generally represented by fewer individuals in nature [32] , [33] and we therefore expect the EN prediction—species clusters each characterized by a distinct mean species body size—to translate into realistic multimodal SADs. To explore this possibility, we run the original model [21] without evolution, using body size as the niche axis. To further support our case for EN, we analyze a real data set documenting a marine phytoplankton assemblage, and explore the relationship between a self-organized community and multimodality in SAD. Basic EN model Running the EN model in its simplest form where species compete along a uniformly suitable niche axis generates a sinusoidal species distribution, showing equally spaced, smooth-looking humps of similar height and separated by valleys ( Fig. 2a ). The relatively steep slopes of this pattern (which can also be analytically derived [34] ) imply that there are more species at the center of the humps and in the valleys than on the slopes. This yields a bimodal SAD in which the mode of rare species corresponds to the valleys on the niche axis, whereas the abundant species come from the core of the humps ( Fig. 2b,c ). 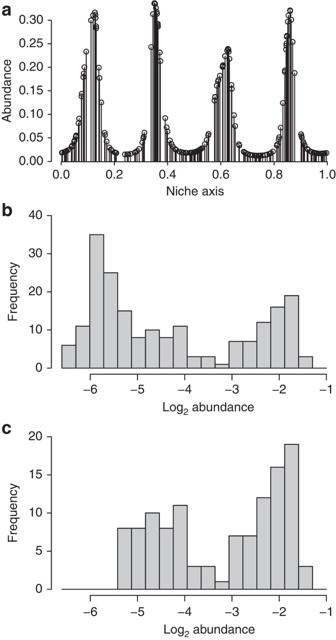Figure 2: Self-organization of species abundances. Simulated competition (no evolution) of species along an initially homogeneous niche axis creates groups of abundant species at self-organized niches, separated by groups of rarer species (a). On a log scale, the SAD for the total set of species is bimodal (b), because there are more species in the 'tops' and the 'valleys' than on the 'slopes' of the sinusoidal landscape in (a). If rare species are assigned higher extinction risks, the number of species in the valleys is thinned out and a relatively smaller mode of rare species emerges (c). Outputs generated a running equation (1) withK=10,r=1,σ=0.15,g=0.02,H=1 and inflow=0.0001. Figure 2: Self-organization of species abundances. Simulated competition (no evolution) of species along an initially homogeneous niche axis creates groups of abundant species at self-organized niches, separated by groups of rarer species ( a ). On a log scale, the SAD for the total set of species is bimodal ( b ), because there are more species in the 'tops' and the 'valleys' than on the 'slopes' of the sinusoidal landscape in ( a ). If rare species are assigned higher extinction risks, the number of species in the valleys is thinned out and a relatively smaller mode of rare species emerges ( c ). Outputs generated a running equation (1) with K =10, r =1, σ =0.15, g =0.02, H =1 and inflow=0.0001. Full size image Varying niche suitability When introducing the more realistic situation of heterogeneous niche suitability in the model ( Fig. 3a ), the simulation output changes to a pattern of valleys and humps whose height and position is something between regular and stochastic ( Fig. 3b ). The partially self-organized humps correspond to suitable niches that each may contain a large number of species. The typical abundance of a species in these clusters can be quite different, depending on how 'good' the niche is and how many species share it. The result in terms of SAD is a multimodal distribution, in which the mode of the least abundant species corresponds to the valleys, whereas the other modes each correspond to a different cluster of species on the niche axis ( Fig. 3c ). Varying niche suitability therefore creates modes of different abundance in the SAD. 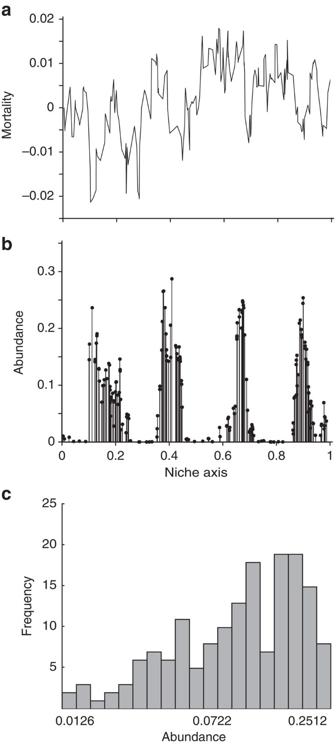Figure 3: Evolution on a pre-existing fitness landscape. (a) Fitness landscape modeled as an additional mortality factor specific to the position on the niche axis. Parameter values used in equation (4) to produce the red noise landscape were:T(0)=0,β=0.005 andλ=20. (b) Position and abundance of individual species after competing and evolving in this landscape (note that this results from the combination of structuring self-organization and irregular pre-existing conditions). Population growth was modeled usingK=10,r=1,σ=0.15,g=0.04,H=1 and inflow=0.00005 in equation (1). Evolution occurred every 10 time steps. (c) Resulting SAD on a log scale for the total set of species. Figure 3: Evolution on a pre-existing fitness landscape. ( a ) Fitness landscape modeled as an additional mortality factor specific to the position on the niche axis. Parameter values used in equation (4) to produce the red noise landscape were: T (0) =0, β =0.005 and λ =20. ( b ) Position and abundance of individual species after competing and evolving in this landscape (note that this results from the combination of structuring self-organization and irregular pre-existing conditions). Population growth was modeled using K =10, r =1, σ =0.15, g =0.04, H =1 and inflow=0.00005 in equation (1). Evolution occurred every 10 time steps. ( c ) Resulting SAD on a log scale for the total set of species. Full size image Body size as a niche descriptor The prediction for the version of the model where we interpret the niche axis as body size (Methods) is a multimodal species size distribution that consists of three clusters of increasingly large and increasingly rare species for this particular parameterization ( Fig. 4a ). Maximum abundance within a cluster of small species is always higher than in a cluster of larger species, but the model also predicts that within a single size cluster, species positioned on the slopes can have markedly lower abundances than more central species. Species belonging to different clusters can therefore have similar abundances, depending on their position ( Fig. 4a,c ). As a result, there is no clean one-to-one relationship between the modes in the SAD and in the self-organized species size distribution. Rather, the consequence in terms of SAD is the presence of multiple modes gathering either species from a single size cluster (that is, central species only, slope species only, or all species) or species from different size clusters that overlap in their abundances ( Fig. 4e ). 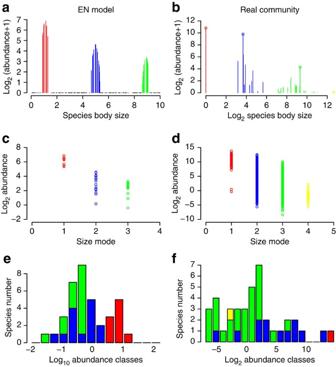Figure 4: Predicted and observed size and abundance distributions. Species distributions predicted under the EN model (left column figures (a), (c) and (e), respectively) and as found in a large empirical phytoplankton data set (right column figures (b), (d) and (f), respectively) are shown. Abundance in the empirical data is expressed in terms of species density. Three modes or clusters of small (red), medium-sized (blue) and large (green) species emerge after 25,000 time steps in the example of community simulated by the EN model (a). This particular output was generated calculating the carrying capacityKifor each species usingKc=900,a=100,Lmax=10,σ=1.5 in equation (6); theKiwere then used in equation (1) withr=1,g=1.5,H=150 and inflow=0 (Methods). The species size distribution for the considered real phytoplankton community (b) shows four distinct species size modes on a log2scale: small (red), medium-sized (blue), large (green) and very large (yellow). Dominant species in each mode are indicated by a circle. In both the simulation output and the real community data, the same color code is preserved in lower panels. Abundance distributions per size mode (c,d) show a degree of overlap between modes. Maximum abundances are always higher for smaller species. Empirical data are weekly abundances over the 12 years of sampling. They decrease with increasing body size and differ significantly among modes (one-way analysis of variance:P<0.001, see main text). Resulting SADs (e,f) show multiple modes comprising species from several size clusters. Figure 4: Predicted and observed size and abundance distributions. Species distributions predicted under the EN model (left column figures ( a ), ( c ) and ( e ), respectively) and as found in a large empirical phytoplankton data set (right column figures ( b ), ( d ) and ( f ), respectively) are shown. Abundance in the empirical data is expressed in terms of species density. Three modes or clusters of small (red), medium-sized (blue) and large (green) species emerge after 25,000 time steps in the example of community simulated by the EN model ( a ). This particular output was generated calculating the carrying capacity K i for each species using K c =900, a =100, L max =10, σ =1.5 in equation (6); the K i were then used in equation (1) with r =1, g =1.5, H =150 and inflow=0 (Methods). The species size distribution for the considered real phytoplankton community ( b ) shows four distinct species size modes on a log 2 scale: small (red), medium-sized (blue), large (green) and very large (yellow). Dominant species in each mode are indicated by a circle. In both the simulation output and the real community data, the same color code is preserved in lower panels. Abundance distributions per size mode ( c , d ) show a degree of overlap between modes. Maximum abundances are always higher for smaller species. Empirical data are weekly abundances over the 12 years of sampling. They decrease with increasing body size and differ significantly among modes (one-way analysis of variance: P <0.001, see main text). Resulting SADs ( e , f ) show multiple modes comprising species from several size clusters. Full size image Empirical example As was expected, abundances decrease with increasing body size ( Fig. 4b,d ; mean abundance mode 1=1809.0±63.8, mean abundance mode 2=90.7±4.5, mean abundance mode 3=1.3±0.2, mean abundance mode 4=0.1±0.02) and a simple one-way analysis of variance shows that they significantly differ among modes ( P <0.001). Hence, species belonging to different size clusters contribute on average to different abundance ranges. Just as in the model predictions, a number of species positioned on the periphery of the two intermediate-size modes have very similar abundances ( Fig. 4b,d ). This is confirmed when looking at the SAD; four modes can be distinguished that all contain a mixture of species belonging to several of the modes identified in the size distribution ( Fig. 4f ). The fact that many SADs appear to be unimodal may indicate that the corresponding communities are not governed by self-organized EN. However, proper testing for multimodality has not been carried out extensively so far, whereas perceived unimodality may also be an artifact of lumping data [3] . The fact that a closer look reveals multimodal patterns in a range of data sets suggests that the existing theories are insufficient to explain true SADs. Obviously, such observed multimodality in natural communities does not necessarily imply that the EN theory is right. As always, even if a pattern is consistent with the theory, it may also be produced by other mechanisms. The most basic conclusion that we may derive from the existence of multiple modes in SADs is that there are distinct groups of species that have a similar abundance (rather than an overall continuum of species abundances). To ponder to what extent the multimodal SADs may be interpreted as evidence for EN, let us consider how the theory comes to the prediction of multimodality, and what might be the alternative explanations. First, EN predicts that there is a group of species that occupies the gaps between the self-organized niches. This group essentially has 'no niche' in the local system and its component species are therefore rare. This concept of outsider species can explain the existence of the distinct group of rare species found in certain observed SADs [10] and relates to a developing body of 'asymmetric' theories. These envisage communities as a collection of distinct groups of species with different characteristics that systematically affect their abundances [35] . In principle, a distinct group of rare visitor species could be added as an extra feature to any traditional SAD theories to produce bimodal patterns. A good example is provided by the neutral theory of diversity, where migrants from the larger metacommunity cause an excess of rare species in the local community they enter and are best described with a logseries SAD, distinct from the lognormal resident distribution [20] , [36] . Asymmetric theories predict multiple abundance modes gathering species with distinct features such as dispersal ability [35] or spatial aggregation [4] . The EN model integrates these asymmetries among species by predicting a default bimodal distribution comprising a rare mode of outsider species and an abundant mode of resident species [28] ( Fig. 2 ). The potential effect of asymmetries on species abundances suggests tracking them will be a necessary first step in studying multimodality empirically. Beyond species asymmetries, the other multiple modes arise in the EN perspective, because there are groups of ecologically similar species that share a (self-organized) niche and are comparable in all aspects, including their abundance. The multiple modes in SADs occur if those self-organized groups differ sufficiently in the typical abundance of the species they contain. As we showed, such a difference in abundance may arise, for instance, if the niches differ in how favorable they are intrinsically, or if species body sizes differ strongly between niches. Another possibility could be that the niches differ widely in the number of species they harbor, as more species sharing a niche should imply lower densities per species. In view of these different possibilities, it seems likely that it will be the rule rather than the exception that self-organized lumps of species will differ in terms of the typical abundance of their constituent species. Therefore, if a community is shaped by EN, it will likely have a multimodal SAD. Even in the absence of EN, one could of course imagine multiple modes to arise due to environmental heterogeneity alone. For example, the textural theory [25] exclusively explains multimodal species size distributions with environmental constraints. In natural systems, EN will never be the only process shaping species abundances, but will always interact with environmental constraints. In a previous work, we have shown that such interaction will likely create a regular, evenly spaced distribution of species abundances in niche space that could not arise from environmental heterogeneity alone [21] . Here we demonstrate that the combined effect of EN and niche suitability could create groups of species with distinct abundances appearing as multiple modes in SADs, where noisy, heterogeneous niche suitability alone would not have necessarily sufficed. Of course, the net effect of the tension between EN and niche suitability will depend on their relative intensity, and particular circumstances may exist where the distribution of resources could exactly counter-balance or completely override the influence of EN. Figure 4 shows an example in which EN is the likely driver of diversity and species abundances [28] yet multiple other processes probably contribute to SAD 'lumpiness' at various spatial, temporal and taxonomic scales, similarly to what is believed to occur in multimodal species body-size distributions [31] . The strength of the EN theory is to provide a universal explanation for how such distinct groups may arise that smoothly integrates the ecological factors and the niche space suitability. In conclusion, although existence of multimodal SADs by itself can obviously not be considered as a proof that EN shapes natural communities, it adds substantially to the credibility of the theory. No other symmetric SAD theory predicts such pattern, and no other species coexistence theory mechanistically links the influence of both species interaction and the environment to diversity structure. It may seem a rather astonishing hypothesis that most species could, in a sense, be more-of-the-same. Indeed, it puts the ecological identity of species in a completely different light [37] . Nonetheless, the case for EN as a force shaping natural communities has become stronger with recent data-based [28] and theoretical [38] , [39] results, and the congruence of its predictions with observed SAD patterns constitutes an independent line of support. Basic EN model The basic EN model is a Lotka–Volterra model, in which species distributed at random along a single niche axis compete for resources. The model is fully described by Scheffer and van Nes [21] , and we only provide the main equations here. The dynamics of species i follows equation (1) where r is the maximum per capita growth rate of species i , N i is the density, K is the carrying capacity and α i,j is the competition coefficient scaling the effect of competitor species j on i . Density-dependent mechanisms regulate the growth of species i through losses up to a maximum g when population density exceeds a threshold H . The inflow parameter mimics the effect of a heterogeneous world, where individuals of species i can enter the simulated local community from other, potentially more favorable patches [40] . The niche of each species is characterized by a normal distribution on the niche axis L . where P i ( L ) is the probability density function for the abundance distribution of species i . μ and σ are the mean and the s.d. of the distribution, respectively. Competition intensity is related to the overlap between the two species' niches, that is, the probability that individuals of i and j are at the same position on the niche axis. Competition coefficient α i,j is calculated as the ratio between the probability of matching an individual of the competing species j and the probability of matching a conspecific. To avoid edge effects, the niche axis is made circular or 'infinite' so that all species have the same number of competitors on their left and right. Varying niche suitability Heterogeneity in niche suitability is modeled by imposing a carrying-capacity landscape to the basic EN model. Practically, this means adding a new mortality term T , modeled as a red noise function of position on the niche axis. where l is a position on the niche axis and ( l −1) is the position that immediately precedes it. Values of l are regularly positioned along the niche axis and mortality T at species positions must be interpolated from them. λ is the period of the noise signal (for red noise: λ >1). T (0) is the value for T at position 0. β quantifies the extent of the noise and C is a normally distributed random number. To show how species can become adapted to pre-existing niches, we implement evolution in the model. This is done by letting species move by a fixed distance of 0.01 on the niche axis every 10 ecological time steps in the direction where competition is less intense. Body size as a niche descriptor We run the original model without evolution [21] taking the niche axis as body size. In this case, we use a 'finite' version of the niche axis, where species at each edge have fewer competitors [21] . If L max is the length of the niche axis, the equation for competition coefficient α i,j becomes: We assume a bell-shaped fitness landscape representing the idea that species at the extremes of the body-size axis face harsher challenges than central species on the more benign central part of the body-size distribution. This is a realistic assumption [31] which guarantees that species on the edges of the niche axis—species that, in the model, experience lower competition—will not take over the simulated community [21] . Note that this smooth unimodal distribution cannot give rise, on its own, to multiple modes of abundance. Where K i is the carrying capacity of species i , K c is the minimum carrying capacity for any species in the community, a is the maximum additional carrying capacity a species can benefit from, μ i is the mean position of species i on the niche axis and L max is the axis length. The EN model deals with biomass abundances, and numerical abundances are simply found by dividing the raw outputs by body size. Empirical example We use an extensive data set documenting species densities in a marine phytoplankton community sampled weekly between 1992 and 2003 in the English Channel ( http://www.westernchannelobservatory.org.uk/l4_phytoplankton ). For the 40 species that are present at all sampling years and constitute the core of the community, the species size distribution shows four distinct modes ( Fig. 4b ), and previous analyses suggest that EN explains this pattern [28] . To assess qualitatively the realism of the EN model, we compare the size structure and the distribution of species abundances from this empirical data set and the predictions from the size-structured EN model. How to cite this article: Vergnon, R. et al . Emergent neutrality leads to multimodal species abundance distributions. Nat. Commun. 3:663 doi: 10.1038/1663 (2012).